Carbon enters silica forming a cristobalite-type CO2–SiO2solid solution Extreme conditions permit unique materials to be synthesized and can significantly update our view of the periodic table. In the case of group IV elements, carbon was always considered to be distinct with respect to its heavier homologues in forming oxides. Here we report the synthesis of a crystalline CO 2 –SiO 2 solid solution by reacting carbon dioxide and silica in a laser-heated diamond anvil cell ( P =16–22 GPa, T >4,000 K), showing that carbon enters silica. Remarkably, this material is recovered to ambient conditions. X-ray diffraction shows that the crystal adopts a densely packed α-cristobalite structure ( P 4 1 2 1 2) with carbon and silicon in fourfold coordination to oxygen at pressures where silica normally adopts a sixfold coordinated rutile-type stishovite structure. An average formula of C 0.6(1) Si 0.4(1) O 2 is consistent with X-ray diffraction and Raman spectroscopy results. These findings may modify our view on oxide chemistry, which is of great interest for materials science, as well as Earth and planetary sciences. Extreme conditions lead to the development of new chemistry [1] , [2] , [3] . Studies are increasingly showing that the known extensive chemical homogeneity among elements of the same group in the periodic table can be extended, in particular, to the lightest elements of the group, which often behave differently under ambient conditions. Until recently, the potential analogy between C and Si in forming extended oxides was very limited. On one hand, there is CO 2 , which is an archetypical gas under normal conditions with carbon in twofold coordination, and the molecule is held together by two strong, double bonds. Molecular CO 2 is the main greenhouse gas. It is one of the main components in the atmosphere of Earth-like planets and it has an important role in volcanic and seismic activity. It is found in ice form in the outer planets and asteroids. It is also used as a supercritical solvent in chemical reactions. Alternatively, SiO 2 is a solid material with Si in either four- or sixfold coordination ( Fig. 1 ). Silica exhibits both amorphous forms and crystalline phases, many of which are important minerals. Silica is also one of the most used technological materials as silica glass and quartz. In many applications, such as in optical waveguides, SiO 2 is also used in solid solutions with GeO 2 , its heavier analogue. Although traditionally perceived as being incompatible, a molecular gas (CO 2 ) and a network solid (SiO 2 ), recent high-pressure experiments have radically altered this view. In fact, CO 2 is found to form non-molecular, amorphous and crystalline silica-like solids above 25–30 GPa composed of CO 4 tetrahedra [4] , [5] , [6] , [7] , [8] , [9] , [10] , [11] , [12] , [13] , [14] . The transformation is linked to the pressure-induced destabilization of the π bonds in CO 2 . However, to date, none of these materials have been recovered at ambient pressure. The possibility that CO 2 –SiO 2 compounds could exist was recently predicted [15] , [16] . The synthesis of such compounds would remarkably add to the chemistry of oxides and would provide an updated view of the periodic table, as well as practical applications. 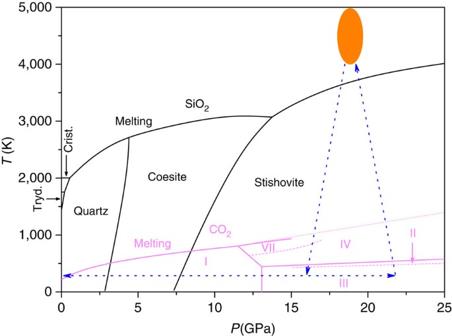Figure 1: Pure SiO2and CO2phase diagrams and P-T path. Black lines: SiO2phase boundaries17. Light magenta, continuous and dotted lines: CO2phase boundaries; light magenta, dashed lines: kinetic boundaries for CO211,18,19,20. Blue dashed arrows and orange ellipse: P-T path followed in this study. All five solid phases of CO2shown are molecular crystals. Non-molecular CO2phases are formed above 25–30 GPa. Crist, cristobalite; Tryd, trydimite. Figure 1: Pure SiO 2 and CO 2 phase diagrams and P-T path. Black lines: SiO 2 phase boundaries [17] . Light magenta, continuous and dotted lines: CO 2 phase boundaries; light magenta, dashed lines: kinetic boundaries for CO 2 [11] , [18] , [19] , [20] . Blue dashed arrows and orange ellipse: P-T path followed in this study. All five solid phases of CO 2 shown are molecular crystals. Non-molecular CO 2 phases are formed above 25–30 GPa. Crist, cristobalite; Tryd, trydimite. Full size image The main challenge in synthesizing such materials is overcoming the incompatibility of the coordination environments of C and Si in solid oxides under any given P-T conditions. The sixfold coordinated phase of SiO 2 , stishovite, is already thermodynamically stable above 7–14 GPa, depending on the temperature [17] , whereas CO 2 is well within the pressure range of stable molecular solids. High pressure and high temperature are mandatory for the formation of carbon in fourfold coordination. Phases with fourfold coordination in CO 2 are only found above 25–30 GPa (see refs 11 , 18 , 19 , 20 and references therein). On the other hand, working pressures cannot be much higher than the transition pressure from coesite to stishovite, 7–14 GPa, in order to limit the chances of forming silicon in sixfold coordination. In order to facilitate the reaction, we used silicalite, a fourfold coordinated SiO 2 zeolite, as the starting phase for SiO 2 , with 5.5 Å diameter micropores (see ref. 21 and references therein) that can readily be filled by atoms and small molecules such as Ar, CO 2 and C 2 H 4 under pressure [22] , [23] , [24] , [25] . The mixture of silicalite and nano-confined CO 2 has a huge interaction surface, and we recently reported a disordered, silicon carbonate phase obtained from these reactants at 18–26 GPa and 600–980 K (ref. 26 ). In silicon carbonate, carbon is threefold coordinated by oxygen and the CO 3 ion has planar structure. Here we present, in contrast to the former material, the synthesis of a CO 2 –SiO 2 solid solution, which is a covalent compound where both Si and C are fourfold coordinated by oxygen. The solid solution is obtained by reacting CO 2 and silica, initially in the form of silicalite, at 16–22 GPa and temperatures in excess of 4,000 K and is characterized by X-ray diffraction (XRD) and Raman spectroscopy. The new phase is recovered at ambient conditions. Synthesis and XRD characterization We loaded the diamond anvil cell (DAC) with a mixture of silicalite and CO 2 and directly heated with a CO 2 laser ( λ =10.6 μm). The sample was thermally insulated by coating the diamond culets with a few micrometre-thick NaCl layers (Methods). We heated the porous silicalite/CO 2 mixture for 30 s at temperatures in excess of 4,000 K at a starting pressure of 21.7 GPa using a laser power density of about 50 KW mm −2 . Under these P-T conditions, both pure SiO 2 and CO 2 are liquid, and the reaction most likely occurs in the liquid state ( Fig. 1 ). After heating, the sample was quenched at room temperature and the pressure was found to be 16 GPa. XRD data were collected at this pressure, at 7 GPa ( Fig. 2 ) and at room pressure on decompression. For all three pressures, in addition to the diffraction peaks of NaCl, a small amount of remaining pure CO 2 (phase I) and Re from the gasket, a series of new strong characteristic sharp diffraction peaks were observed. These diffraction peaks could readily be indexed using a tetragonal unit cell with a c / a ratio between 1.283 at 16 GPa and 1.303 at 0 GPa ( Fig. 2 and Table 1 ). Unfortunately, the diffracted intensities were not reliable as they do not correspond to a randomly oriented powder, but to only several well-crystallized particles formed at the very high temperature used to obtain this new material. We were thus only able to refine the unit cell parameters. The observed systematic absences are consistent with the P 4 1 2 1 2 space group of the α-cristobalite structure, and the indexation of the strongest, low-angle diffraction peaks is the same as that of α-cristobalite SiO 2 (ref. 27 ). This space group implies that the Si and C atoms are randomly distributed on the 4 a Wyckoff positions in a disordered manner and corresponds to the statistically average structure of the solid solution. In the present case, the c / a values are lower than those of pure SiO 2 which decrease from 1.391 at room pressure to 1.3329 at 9.1 GPa (refs 28 , 29 ), owing to the more compact structure of the new material. The unit cell volume of this new α-cristobalite-type phase is 6% lower than that of pure SiO 2 at 7 GPa and 26% lower at ambient pressure. This is entirely consistent with the incorporation of much smaller carbon atoms, which replace silicon in the α-cristobalite-type structure, leading to a collapse of the oxygen sublattice. If one interpolates between the ambient pressure experimental unit cell volume of SiO 2 ( V =171.42 Å 3 ) (ref. 28 ) and the theoretical volume of metastable α-cristobalite-type CO 2 ( V =88.04 Å 3 ) (ref. 7 ) using Vegard’s law, the chemical composition of the solid solution ( V =127.61 Å 3 ) can be estimated to be ∼ C 0.5 Si 0.5 0 2 . The c / a values for this new phase are lower than those of pure SiO 2 α-cristobalite at high pressure after significant collapse of the pure SiO 2 structure, and are essentially equivalent to that of the rutile-type oxygen sublattice, which can be described using the same unit cell with a c / a ratio of 1.288 (ref. 30 ). This collapse to a dense oxygen sublattice can explain the very small variation in volume with pressure observed for this phase. Although the data points are not sufficient to be fitted to an equation of state and the remaining molecular CO 2 is a soft solid and not truly hydrostatic (maximum pressure variations of ±7% were observed over the whole sample surface; note that the pressure was measured at the same spot as the diffraction pattern with the 2-μm diameter X-ray beam to minimize errors), a bulk modulus of the order of 240 GPa is consistent with the experimental data. If one describes rutile-type silica, stishovite, using the same unit cell, the c / a ratio varies from 1.276 at ambient pressure [31] to 1.298 at 55 GPa (ref. 32 ). The present result is also consistent with theoretical studies of the α-cristobalite—stishovite phase transition mechanism [33] , [34] , which predict that the transition occurs in two steps: first the α-cristobalite-type structure collapses such that the oxygen sublattice is equivalent to that in the rutile-type structure, and then the cations migrate to octahedral sites. The present material corresponds at high pressure to end of the first step and it is most probably retained owing to the significant amount of carbon in the structure, which does not have a tendency to pass into octahedral coordination. In the case of the CO 2 –SiO 2 solid solution, an α-cristobalite structure is obtained rather than a collapsed I 2 d cristobalite structure, as in CO 2 phase V , due to the presence of larger Si 4+ cations. The collapsed cristobalite structure is characteristic of materials containing small cations, typically B 3+ , C 4+ and P 5+ (refs 13 , 30 , 35 , 36 ). 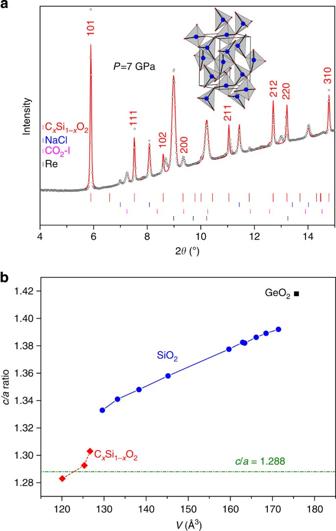Figure 2: XRD pattern and structure and unit cell volume dependence of thec/aratio of the solid solution. (a) Experimental (dots) and calculated (Le Bail fit—red line) XRD patterns at 7 GPa. Vertical bars: diffraction angles of the α-cristobalite (P41212) solid solution, CO2-I from unreacted CO2, NaCl, used for thermally insulating the sample, and Re from the gasket. Inset: structure of the solid solution (C/Si atoms in blue and O atoms in red). (b)c/aratio as a function of the unit cell volume for the α-cristobalite-type solid solution and pure α-cristobalite-type SiO228,29and GeO245, respectively. The value ofc/a=1.288 corresponds to a rutile-type oxygen sublattice. Figure 2: XRD pattern and structure and unit cell volume dependence of the c / a ratio of the solid solution. ( a ) Experimental (dots) and calculated (Le Bail fit—red line) XRD patterns at 7 GPa. Vertical bars: diffraction angles of the α-cristobalite (P4 1 2 1 2) solid solution, CO 2 -I from unreacted CO 2 , NaCl, used for thermally insulating the sample, and Re from the gasket. Inset: structure of the solid solution (C/Si atoms in blue and O atoms in red). ( b ) c / a ratio as a function of the unit cell volume for the α-cristobalite-type solid solution and pure α-cristobalite-type SiO 2 [28] , [29] and GeO 2 [45] , respectively. The value of c / a =1.288 corresponds to a rutile-type oxygen sublattice. Full size image Table 1 Lattice parameters (Å) and c / a ratio for the solid solution with the P 4 1 2 1 2 structure. Full size table Raman spectroscopy characterization Raman spectroscopy was essential to determine the nature of the chemical bonds in the solid solution and to check for other possible materials present in the sample region. In addition to signatures of the solid solution ( Fig. 3 ) and of unreacted, molecular CO 2 (see also XRD), we found some microcrystalline/amorphous graphite with broad peaks in the 1,300–1,600 cm −1 frequency range, which is consistent with the blackish aspect of part of the sample and confirms that some of the initial CO 2 precursor was indeed dissociated at high temperature. Dissociation of CO 2 under high P-T conditions was reported by other authors (ref. 19 and references therein). 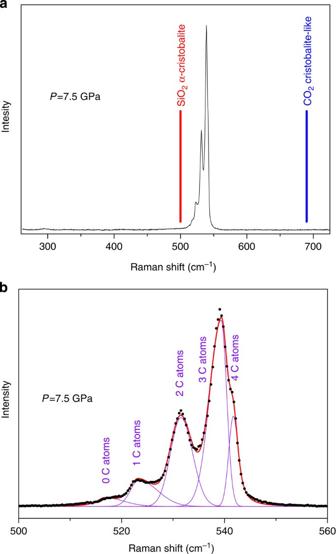Figure 3: Selected Raman spectrum of the solid solution. (a) Full view, with frequency positions observed for similar tetrahedral structures of pure SiO2(α-cristobalite, extrapolated to 7.5 GPa37) and non-molecular CO2(experimental collapsed β-cristobalite like11,13,18). (b) Zoom of the fine structure of the peak (dots) fitted to five peaks (violet for the single components and red for the sum), which we assign to unit cells containing different numbers of C and Si atoms, respectively, that is, unit cell content: CnSi4−nO8, wheren=0, 1, 2,…4. Figure 3: Selected Raman spectrum of the solid solution. ( a ) Full view, with frequency positions observed for similar tetrahedral structures of pure SiO 2 (α-cristobalite, extrapolated to 7.5 GPa [37] ) and non-molecular CO 2 (experimental collapsed β-cristobalite like [11] , [13] , [18] ). ( b ) Zoom of the fine structure of the peak (dots) fitted to five peaks (violet for the single components and red for the sum), which we assign to unit cells containing different numbers of C and Si atoms, respectively, that is, unit cell content: C n Si 4− n O 8 , where n =0, 1, 2,…4. Full size image The spectrum of the C x Si 1-x O 2 solid solution is dominated by a sharp peak with fine structure at around 540 cm −1 , which we easily assign to deformation modes of the tetrahedra. In fact, this peak lies in between the analogous, strong peaks of pure α-cristobalite SiO 2 (ref. 37 ) and cristobalite-like CO 2 (refs 11 , 13 , 18 ), respectively. This mode displays higher frequency for the solid solution than for α-cristobalite SiO 2 because of the smaller reduced mode mass and the stronger bond strength with respect to that of pure SiO 2 . On the other hand, the frequency is lower than in non-molecular CO 2 , where the reduced mode mass is smaller and the bond strength is stronger. It has been recently found that amorphous silicon oxycarbide materials of potential interest for planetary interiors can be synthesized as a result of carbon substitution for oxygen in silicates [38] . This kind of material includes Si–C chemical bonds, which typically exhibit intense Raman peaks at frequencies >750–800 cm −1 (ref. 39 ). As we do not observe similar peaks, carbon substitution for oxygen rather than for silicon is ruled out in our solid solution. We also rule out the presence of silicon carbonate [26] in the present material, which would exhibit much higher frequencies than those reported in our Raman spectrum. In addition, silicon carbonate, in contrast to our solid solution, was not recovered to ambient conditions. A remarkable insight now comes from the analysis of the fine structure of the peak ( Fig. 3b and Table 2 ). This peak was fit to five slightly asymmetric components that we assign to the same vibrational mode of unit cells containing different numbers of C and Si atoms, respectively, that is, unit cell content: C n Si 4− n O 8 , where n =0, 1, 2,…4. Therefore, we have the lowest frequency component that corresponds to unit cells with 0 C and 4 Si atoms, up to the highest frequency component corresponding to unit cells with 4 C and 0 Si atoms. The number of components in the Raman peak, five, arises from individual cells with the five different possible contents, and the relative intensities are because of the statistical amount of each type of unit cell content linked to the chemical composition of the solid solution. Therefore, the statistical average of the n index, n average , will not be an integer, but rather a real number ranging between 0 and 4. The relative intensities of the five Raman components ( Table 2 ) can then be used to estimate the stoichiometry of the C x Si 1− x O 2 solid solution. This result can be compared with the analogous value obtained based on the unit cell volume from the XRD analysis. The statistical distribution of the number n obtained in this way yields: n average =2.8(8), where the statistical error is given by the s.d. of the distribution. The spatial dependence of n average was also checked over the whole sample surface, and the changes in this quantity have been found to be negligible with respect to the statistical error estimated at each single point. Therefore, as we have four cations in the generic unit cell, the average value for the composition x will be: x average = n average /4=0.7(2), giving a chemical formula for the solid solution of C 0.7(2) Si 0.3(2) O 2 . This result is consistent with the chemical formula obtained from the XRD analysis, although higher in C content, and an average chemical formula of C 0.6(1) Si 0.4(1) O 2 agrees with both the XRD and the Raman results. We note that the high carbon content identified by the combination of these two methods is consistent with the strong decrease in c / a lattice parameter ratio with respect to pure SiO 2 at a volume of about 130 Å 3 in the relationship between c / a and unit cell volume for α-cristobalite-type structures ( Fig. 2b ). The small size of carbon results in a collapse of the structure. The decrease in c / a is of a similar order of magnitude as that between GeO 2 and SiO 2 . Table 2 Relevant parameters of the peaks fitted to the Raman spectrum of the solid solution. Full size table The present study using a combination of XRD and Raman spectroscopy clearly shows that a solid solution between CO 2 and SiO 2 with an α-cristobalite-type structure can be obtained under high P-T conditions. The P-T ( P =16–22 GPa, T>4,000 K) conditions for the formation of such a solid solution correspond to a compromise between the respective stabilities of three- and fourfold coordination in CO 2 and four- and sixfold coordination in SiO 2 . The formation of the solid solution enables one to retain a metastable hard solid based on CO 4 tetrahedra down to ambient conditions owing to the incorporation of a quantity of silicon atoms. A new oxide chemistry is now possible in which silicon atoms can be replaced by carbon in silica and even silicates. This chemistry can give rise to a unique class of materials with novel physical properties, a class of hard, light, carbon-rich oxides, metastable at ambient conditions, with high thermal conductivity and application-tailored index of refraction. Such carbon-substituted materials may also be relevant for Earth and planetary sciences. Powder XRD methods Angle-dispersive powder XRD patterns were obtained on the ID27 beam line at the European Synchrotron Radiation Facility (ESRF) using a monochromatic beam ( λ =0.3738 Å) and a MAR165 CCD detector. The nominal size of the X-ray focal spot was 2 μm. The diffraction patterns were analysed and integrated using the FIT2D programme [40] . The Le Bail fit to the XRD data was performed using the programme Fullprof [41] . Raman spectroscopy methods Raman spectra (2–3-μm focal spot) were measured using the 647.1 nm line of a Kr + laser as the excitation source, and the setup is described elsewhere [13] . The spatial uniformity of the sample was checked using 4 μm step meshes, and the typical spectrum of the solid solution ( Fig. 3 ) was found over about 50% of the sample surface. Synthesis and high-pressure methods Hydrophobic silicalite-1-F was obtained from SOMEZ. A DAC was used for the high-pressure experiments. CO 2 was loaded in the DAC (IIa diamonds were used, as they are transparent for the CO 2 laser) in the liquid phase at −20 °C and 30 bar together with powdered silicalite. The diameter (thickness) of the rhenium gasket used as a sample chamber after DAC loading was 80 μm (40 μm). Diamond culets were coated by a few micrometre-thick NaCl layers in order to thermally insulate the sample during the laser heating. Laser heating was performed for 30–60 s in different points of the sample with a CO 2 laser ( λ =10.6 μm), and temperature was measured by optical pyrometry [42] . The maximum laser power and beam spot were of 150 W and 30–40 μm, respectively. The NaCl-coating layers were also used for measuring the pressure during the XRD experiment based on the equation of state of NaCl [43] . The pressure shift of the Raman diamond peak was used for measuring the pressure during the Raman measurements [44] . How to cite this article: Santoro, M. et al. Carbon enters silica forming a cristobalite-type CO 2 –SiO 2 solid solution. Nat. Commun. 5:3761 doi: 10.1038/ncomms4761 (2014).